Integrated optical auto-correlator based on third-harmonic generation in a silicon photonic crystal waveguide The ability to use coherent light for material science and applications is linked to our ability to measure short optical pulses. While free-space optical methods are well established, achieving this on a chip would offer the greatest benefit in footprint, performance and cost, and allow the integration with complementary signal-processing devices. A key goal is to achieve operation at sub-watt peak power levels and on sub-picosecond timescales. Previous integrated demonstrations require either a temporally synchronized reference pulse, an off-chip spectrometer or long tunable delay lines. Here we report a device capable of achieving single-shot time-domain measurements of near-infrared picosecond pulses based on an ultra-compact integrated CMOS-compatible device, which could operate without any external instrumentation. It relies on optical third-harmonic generation in a slow-light silicon waveguide. Our method can also serve as an in situ diagnostic tool to map, at visible wavelengths, the propagation dynamics of near-infrared pulses in photonic crystals. In the last decade, silicon photonics has enabled the development of a wide range of integrated all-optical signal-processing devices [1] on CMOS-compatible chips that have achieved an impressive array of new capabilities, from switching and demultiplexing at unprecedented speeds [2] , to parametric gain [3] , Raman lasing [4] , optical logic [5] , regeneration [6] , terahertz bandwidth radio frequency (RF) spectrometers [7] , temporal optical cloaking [8] and many others. However, an integrated chip-based pulse measurement device that is capable of single-shot measurements, without the need for a reference pulse, averaging or some external instrumentation that is difficult to integrate, such as an optical spectrum analyser or a long tunable delay line, is still lacking. While several groups have replicated all-optical techniques on a chip [9] , [10] , [11] , [12] that are well established in free space or fibre optics, such as auto-correlation, frequency-resolved optical gating (FROG) or temporal sampling, with obvious benefits in footprint, energy consumption and performance, all of the demonstrations fall short in one of the aforementioned points. A fully integrated pulse measurement technology is nonetheless highly attractive, enabling the complete integration of pulse generation, optical processing and measurement schemes on a single chip. This would provide an extremely flexible integrated processing platform, in particular, in conjunction with integrated pulse shaping [13] or arbitrary waveform generation [14] . The silicon-on-insulator technology offers many attractive features for nonlinear optics [1] . Its high refractive index allows tight confinement of light within nanowires that, combined with the high silicon Kerr nonlinearity ( n 2 ), has yielded extremely high nonlinear parameters ( γ ) of ~300 W −1 m −1 , that is, four–five orders of magnitude larger than in silica fibres ( γ = ωn 2 / cA eff , where A eff is the effective area of the waveguide, c is the speed of light and ω is the optical signal frequency). Furthermore, silicon-on-insulator has proven to be a powerful platform for enhancing nonlinear optical effects over short propagation distances (well below 1 mm) by increasing the optical beam intensity via so-called ‘slow light’ in planar photonic crystal (PhC) waveguides [15] , [16] . In contrast to resonant cavities that only accommodate very limited optical bandwidth, advanced slow-light PhC waveguide designs have been able to offer both wide bandwidth and relatively low dispersion, that is, ‘flatband’ operation [17] with relatively low propagation losses [18] . This is critical for processing short optical signals since slow light is otherwise associated with the dispersive band edge of PhC waveguides, which tends to strongly broaden and distort short optical pulses [19] . By enhancing the effective Kerr nonlinearity in this manner, slow-light planar PhC waveguides have yielded much more compact devices [20] , [21] , [22] , [23] , [24] that are compatible with high-speed signals [24] , [25] . In particular, slow-light-enhanced optical third-harmonic generation (THG) was reported in silicon PhC waveguides [22] and subsequently exploited to monitor the quality of 640 Gb s −1 optical signals [24] . Here, we report a novel application of THG in slow-light silicon PhC waveguides to achieve single-shot temporal measurements via the auto-correlation of picosecond optical pulses. The visible-light signal emitted off the chip effectively maps the temporal characteristics of the near-infrared pulse into spatial dimensions, which can easily be acquired with an out-of-plane camera or detector array. A number of integrated all-optical techniques have already been reported [9] , [10] , [11] , [12] , [26] , [27] to achieve time-resolved measurements of ultra-high-speed optical signals as an alternative to expensive, bulk-optics-based, commercial optical auto-correlators. These include time-lens temporal imaging on a silicon chip [9] , [26] , and for phase-sensitive pulse measurements, waveguide-based FROG [10] , [27] and a novel variation of spectral phase interferometry for direct electric-field reconstruction (SPIDER) [11] . In contrast to these techniques, our demonstration neither relies on off-chip optical spectrum analysers [9] , [11] , [26] , nor on a complicated numerical extraction algorithm [11] . Further, no reference pulse or long tunable delay lines [10] , [12] are required, and unlike sampling approaches [10] , there is no need to average over many pulses. The simple and extremely compact (96 μm long) device reported here opens the door to the realization of the first fully integrated all-optical device capable of single-shot high-speed optical signal diagnostics in the near-infrared telecommunications window. The technique also produces the equivalent of time-of-flight measurements of picosecond pulses as they propagate through slow-light photonic crystal waveguides. This capability provides a powerful in situ diagnostic tool that allows us to obtain new insights into the propagation dynamics of a slow-light pulse and to directly extract its group velocity. Device principle The principle of operation for the auto-correlator and the experimental set-up for characterizing the device performance are shown in Fig. 1 . When near-infrared pulses (~1,550 nm) propagate along the waveguide independently from either side, they produce THG, that is, visible light at the third-harmonic (TH) wavelength (~530 nm), due to the ultra-fast third-order optical nonlinearity in the silicon PhC waveguide [22] . The efficiency of this process is significantly enhanced by the large (typically ~30) group index in these slow-light waveguides [22] . The spatial profile of THG-induced visible light along the waveguide is relatively uniform for each pulse separately, but when the counter-propagating pulse replicas are made to overlap within the PhC waveguide, an additional THG component—referred to as cross-THG—produces a spatially varying intensity profile along the slow-light PhC waveguide. This stationary pattern of visible light is proportional to the interference of the two pulse replicas—that is, it effectively maps the temporal auto-correlation of the pulse into space in a way similar to the free-space optics scheme demonstrated in a SHG-based bulk crystal with kilowatt peak power pulses [28] . As represented in Fig. 1b , imaging this spatial intensity profile then yields the temporal auto-correlation of the pulse, potentially for a single pulse, or so-called ‘single-shot’ operation—a key advantage over other approaches that are sampling based, such as FROG, and rely on averaging over thousands or even millions of pulses. 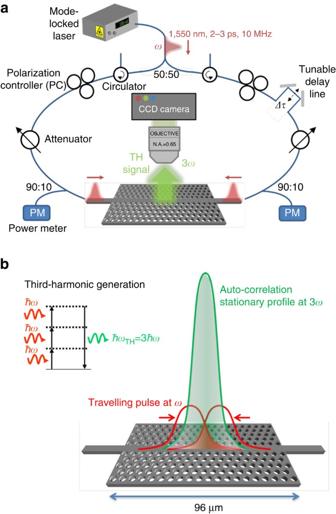Figure 1: Principle of the auto-correlation device and set-up used to demonstrate its operation. (a) Set-up used to probe the photonic crystal waveguide in a counter-propagating configuration. (b) Schematic of the THG-based auto-correlation technique where two counter-propagating pulse replicas at the fundamental frequency interact to generate a stationary spatial profile at the third-harmonic frequency (visible wavelength) directly related to the pulse auto-correlation trace. Figure 1: Principle of the auto-correlation device and set-up used to demonstrate its operation. ( a ) Set-up used to probe the photonic crystal waveguide in a counter-propagating configuration. ( b ) Schematic of the THG-based auto-correlation technique where two counter-propagating pulse replicas at the fundamental frequency interact to generate a stationary spatial profile at the third-harmonic frequency (visible wavelength) directly related to the pulse auto-correlation trace. Full size image Figure 1a shows the experimental configuration for characterizing the device. Optical pulses ~2.5 ps wide from a tunable mode-locked fibre laser are split into two and launched into opposite ends of the PhC waveguide (see Methods). The relative delay between the two counter-propagating pulses can be adjusted to control whether or not the pulses overlap in time while propagating in the PhC waveguide. A high numerical aperture (NA) (0.65) objective and a CCD visible wavelength camera are used to collect and image the TH signal emitted along the PhC waveguide from the top of the chip. The spatial profile of the TH signal, imaged onto the CCD detector, thus directly converts the temporal profile of the pulse auto-correlation into a spatial intensity profile. Note that while the two arms of the set-up include numerous off-chip components to control polarization, circulators and attenuators to balance the optical power of the two beams launched from either side, as well as a tunable delay line in one arm to match the optical path lengths, most if not all of these components are employed just to provide a clear proof of principle of the device operation. They could all readily be avoided with the simple use of an integrated 3 dB splitter on-chip as was successfully demonstrated for SWIFT-integrated spectrometers (stationary-wave integrated Fourier-transform spectrometry) [29] . 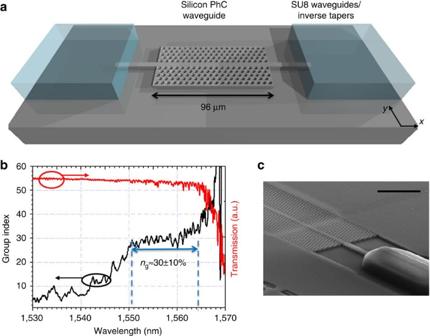Figure 2: Device architecture and characteristics. (a) Schematic of the chip including the silicon slow-light photonic crystal waveguide suspended in air, and connected to SU8 waveguides and inverse tapers for light coupling. (b) Group index dispersion and associated transmission of the photonic crystal waveguide. (c) Scanning electron image of the device. The scale bar on the top right hand side corresponds to 5 μm. Device architecture Figure 2 shows a schematic of the slow-light PhC waveguide along with an s.e.m. picture of the device and the group index versus wavelength measured by interferometric techniques [30] . The device consists of a 96-μm-long silicon PhC waveguide in a 220-nm-thick membrane suspended in air (see Methods). It is connected on both sides to silicon ridge waveguides terminated by inverse tapers and embedded in polymer waveguides to provide a total insertion loss of ~−9.5 dB (fibre-to-fibre). The PhC waveguide is created from a triangular lattice of air holes (period ~404 nm, radius ~116 nm), with one row omitted along the ΓK direction and the first surrounding rows laterally shifted to engineer the waveguide dispersion [17] . Unlike the highly dispersive slow-light mode associated with the band edge of typical PhC waveguides [19] , here the fundamental mode is engineered to display both low group velocity and low dispersion. As displayed in Fig. 2b , the resulting group velocity in this device is ~ c /30 within 10% over a bandwidth exceeding 15 nm, that is, readily compatible with the use of high-speed Tb s −1 signals [24] . Figure 2: Device architecture and characteristics. ( a ) Schematic of the chip including the silicon slow-light photonic crystal waveguide suspended in air, and connected to SU8 waveguides and inverse tapers for light coupling. ( b ) Group index dispersion and associated transmission of the photonic crystal waveguide. ( c ) Scanning electron image of the device. The scale bar on the top right hand side corresponds to 5 μm. 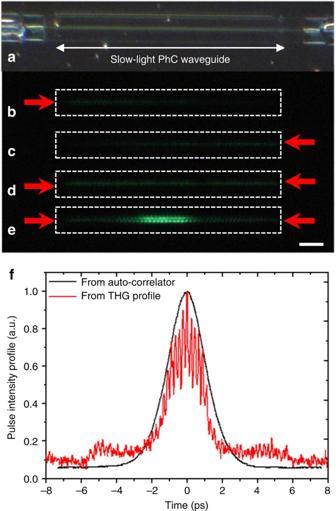Figure 3: On-chip THG-based pulse auto-correlation measurements. Top visible CCD images of the PhC waveguide (displayed on (a) under illumination) showing the TH light generated on exciting the waveguide at 1,548 nm from the left only (b), the right only (c) and from both sides with the off-chip delay line set to 0 ps (d) and 137 ps (e). The dotted white line highlights the boundary of the slow-light PhC waveguide where the green light is emitted and the scale bar at the bottom right represents 10 μm. (f) Pulse intensity profile recovered from the THG profile (red) on the CCD image (e) and measured with a commercial auto-correlator (black). Full size image Pulse auto-correlation measurements Figure 3 shows a series of images recorded on the CCD camera when pulses at 1,548 nm are launched into the waveguide from one side only ( Fig. 3b,c ) and from both sides with the delay line adjusted so that the two pulses overlap either off-chip ( Fig. 3d ) or in the middle of the PhC waveguide ( Fig. 3e ). For cases where the pulses do not overlap on the chip, the TH green light signal is relatively uniform with a low power level, which effectively provides a relatively weak and uniform auto-correlation background. By contrast, when the delay is adjusted such that the pulses overlap inside the PhC waveguide, the average power of TH light is much larger and the associated spatial intensity profile exhibits a stationary Gaussian-like shape centred around the middle of the PhC waveguide. This pattern results from cross-THG produced from the interaction between the left and right near-infrared pulses in the PhC waveguide. From the spatial profile of the TH-power extracted from the CCD image, we retrieve the temporal pulse intensity profile, taking into account the ~ c /23 group velocity at which the 1,548 nm wavelength pulses propagate in the PhC waveguide (see Methods). This intensity profile is compared in Fig. 3f with that measured at the output of the laser using a commercial second-harmonic-generation-based auto-correlator. In this time-resolved plot, the physical boundaries of the slow-light PhC waveguide coincide with the points at around ±6 ps, outside of which no TH light is recorded, only noise. The full-width at half maximum (FWHM) inferred from the THG profile is ~2.4 ps, agreeing relatively well with 2.6 ps obtained via the commercial auto-correlator. The deviation at both edges of the profile is due to the residual TH average signal generated when the two pulses are launched into the waveguide separately from either side. Although it is lower than for SHG-based auto-correlation [31] , this background does reduce the signal-to-noise ratio. In our case though, it can be completely suppressed by using appropriate spatial filtering. Figure 3: On-chip THG-based pulse auto-correlation measurements. Top visible CCD images of the PhC waveguide (displayed on ( a ) under illumination) showing the TH light generated on exciting the waveguide at 1,548 nm from the left only ( b ), the right only ( c ) and from both sides with the off-chip delay line set to 0 ps ( d ) and 137 ps ( e ). The dotted white line highlights the boundary of the slow-light PhC waveguide where the green light is emitted and the scale bar at the bottom right represents 10 μm. ( f ) Pulse intensity profile recovered from the THG profile (red) on the CCD image ( e ) and measured with a commercial auto-correlator (black). 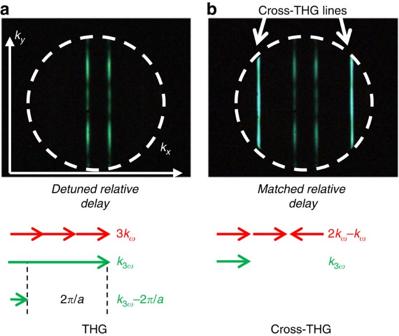Figure 4: Fourier optics analysis of the auto-correlation trace at the third-harmonic frequency. Fourier-space images of the signal generated at the third-harmonic visible wavelength, when the counter-propagating pulses overlap off-chip (a) or into the photonic crystal waveguide (b). In the latter case, two additional lines appear in thek-space, associated with cross-THG between two (respectively one) left and one (respectively two) right photons. The conservation of photon momentum in the direction of the waveguide (quasi-phase matching alongkx) for the THG and cross-THG processes are represented below the images, explaining the different lines observed in both cases. Full size image Figure 4 illustrates the possibility to implement such a spatial filtering scheme by imaging the TH output in the Fourier plane [32] , [33] . Additional cross-terms in k -space (extreme side lines on Fig. 4b ) are observed when the optical pulses overlap in the PhC waveguide. These are due to the interaction of two left (respectively right) fundamental photons with one right (respectively left) photon to generate one TH photon, instead of classical THG where all fundamental photons come from the same side. The momentum conservation of the photons involved in the nonlinear process are represented in Fig. 4a,b for THG and cross-THG, explaining the different lines observed in Fig. 4 (at ±(3 k ω −2 π / a ) for THG and ± k ω for cross-THG). Note that unlike free-space schemes that typically require accurate angle tuning, this quasi-phase matching for cross-THG is naturally ensured by the planar PhC waveguide geometry, independently of the frequency of the fundamental beam [32] . In principle, spatially filtering out the k -components closer to the optical axis would eliminate THG induced by the separate pulses and yield a background-free auto-correlation trace. As expected, the cross-THG signal observed in the Fourier plane in Fig. 4b is more intense than that of the THG. Indeed, the overall intensity of the combined left and right pulses is larger than their separate intensities, while the THG process scales with the cube of the intensity at the fundamental frequency. Note, however, that for our specific waveguide geometry, the fundamental mode wavevector ( k ω ≈0.3 [2 π / a ]) positions the cross-THG lines ( k 3 ω =± k ω ) off-centre of the objective NA (represented by the dashed white circle in Fig. 4 ). This decreases the collection of the relevant cross-THG relative to the separate THG process, effectively increasing the THG background superimposed on the auto-correlation trace observed in the real TH images. Figure 4: Fourier optics analysis of the auto-correlation trace at the third-harmonic frequency. Fourier-space images of the signal generated at the third-harmonic visible wavelength, when the counter-propagating pulses overlap off-chip ( a ) or into the photonic crystal waveguide ( b ). In the latter case, two additional lines appear in the k -space, associated with cross-THG between two (respectively one) left and one (respectively two) right photons. The conservation of photon momentum in the direction of the waveguide (quasi-phase matching along k x ) for the THG and cross-THG processes are represented below the images, explaining the different lines observed in both cases. Full size image In addition to providing the nonlinear enhancement sustaining the THG process, slow-light propagation spatially compresses the pulse [34] , providing the basis for more compact devices. Using the device in regions having different group velocities also enables the measurement of a wide range of pulse durations within a very short waveguide by effectively adjusting the sensitivity and temporal resolution of the device. We investigate the effect of group velocity on the device performance, by studying the behaviour of the device in a regime where the group velocity of the fundamental mode varies almost linearly, by a factor of four, from c /8 to c /30 between 1,540 and 1,550 nm (see Fig. 2b ). 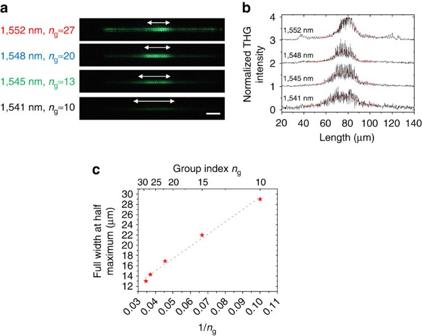Figure 5: Impact of the light pulse group velocity on the auto-correlation device performance. (a) Top visible images of the waveguide obtained when launching pulses with similar durations at different wavelengths, corresponding to different group velocities; the scale bar at the bottom right represents 10 μm. (b) Normalized TH signals across the photonic crystal waveguide length (shifted vertically for clarity). (c) Displays the full-width at half maximum of the TH intensity profile, as fitted by a Gaussian (red lines on (b)) versus the inverse of the group index at the different wavelengths probed. The data shown as red stars follow a linear trend (dotted line). Figure 5a shows the measured TH spatial profiles obtained when launching pulses with similar durations tuned to slightly different wavelengths. We fit the TH patterns with Gaussian curves (see Fig. 5b ) and plot the associated FWHM in Fig. 5c , which follows the expected linear trend with the inverse of the group index [34] . We thus directly observe the spatial pulse compression effect for decreasing group velocities. Selecting the waveguide group velocity can therefore be used to tune the auto-correlator performance, through adjustment of the device calibration, temporal resolution and sensitivity (see Table 1 ). For instance, with the present ~100-μm-long slow-light waveguide, pulses with a maximum duration of 17 ps can be readily measured with a resolution greater than ~69 fs, while a resolution better than 20 fs is available at a lower ( c /8) group index. On the short-range side, pulses as short as 550 fs can be measured, limited here by the dispersion in the flat-band slow-light window of the waveguide under test. Figure 5: Impact of the light pulse group velocity on the auto-correlation device performance. ( a ) Top visible images of the waveguide obtained when launching pulses with similar durations at different wavelengths, corresponding to different group velocities; the scale bar at the bottom right represents 10 μm. ( b ) Normalized TH signals across the photonic crystal waveguide length (shifted vertically for clarity). ( c ) Displays the full-width at half maximum of the TH intensity profile, as fitted by a Gaussian (red lines on ( b )) versus the inverse of the group index at the different wavelengths probed. The data shown as red stars follow a linear trend (dotted line). Full size image Table 1 Performance of the slow-light waveguide-based auto-correlator device. Full size table Group velocity measurements A novel and significant feature of our approach is that, conversely, it can serve as a diagnostic tool to directly measure and study the near-infrared pulse propagation and group velocity in the slow-light regime of a PhC waveguide—that is, in a regime where measurements become difficult. This can be achieved by sweeping the off-chip delay line and tracking the peak of the TH profile along the waveguide. 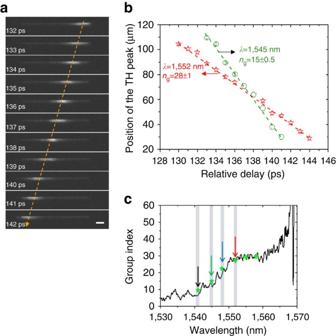Figure 6: Time-of-flight group velocity measurements using the THG-based auto-correlation device. (a) Top visible images of the TH signal for various relative delays between the right and left arms adjusted off-chip (λ=1,548 nm,ng≈20); the scale bar represents 10 μm. (b) Position of the TH peak intensity centre along the waveguide versus the relative delay for a signal wavelength of 1552, nm (red stars) and 1545, nm (green circles). The group velocity at which the pulse propagates can be inferred from the slope of the linear fit (dashed line) to these curves. (c) Group index measured from the TH images (green stars) overlaid on the waveguide dispersion that was measured by interferometric methods. The coloured arrows correspond to the four different wavelengths probed onFigs 5a,band6a, while the grey areas indicate the bandwidth associated with the 2.5 ps pulses. Figure 6a shows the equivalent of time-of-flight measurements, with a series of snapshots of the spatial (thus temporal) profile of the pulse as it ‘propagates’ across the chip. The series of images is obtained by varying the relative temporal delay between the two incident pulses in the right and left arm, within 10 ps, which effectively changes the location at which the two pulses meet within the PhC waveguide. From this, we can extract the group index for different wavelengths, in a way that is much more direct and easier than traditional interferometric measurements, which typically require high stability and data post treatment. Figure 6b shows the spatial shift of the TH profile versus temporal delay at two different wavelengths (1,545 and 1,552 nm), corresponding to two different group velocities. Since the TH peak location corresponds to the point at which the two pulses overlap within the PhC waveguide, the group index can be inferred, without any fit parameter or assumption, from the slope of these linear curves, resulting in an n g =15 and 28 at the two probed wavelengths (see Methods). Figure 6c presents the mapped group index measured at six different wavelengths, overlaid with the group velocity dispersion obtained by interferometric means [30] , showing good agreement between the two. The measurement of the group velocity and the slow-light-induced spatial compression of the pulse are just two examples of in situ information related to the pulse propagation that can be retrieved. Additional key information relates to the capability of the pulse to preserve its integrity at low speeds, where the ballistic regime has been questioned in the presence of disorder [35] , [36] . This time-to-space mapping technique combined with a tunable delay line therefore enables the direct observation of the pulse propagation dynamics as an alternative to powerful but relatively slow and complex heterodyne NSOM techniques [34] , [37] . Figure 6: Time-of-flight group velocity measurements using the THG-based auto-correlation device. ( a ) Top visible images of the TH signal for various relative delays between the right and left arms adjusted off-chip ( λ =1,548 nm, n g ≈20); the scale bar represents 10 μm. ( b ) Position of the TH peak intensity centre along the waveguide versus the relative delay for a signal wavelength of 1552, nm (red stars) and 1545, nm (green circles). The group velocity at which the pulse propagates can be inferred from the slope of the linear fit (dashed line) to these curves. ( c ) Group index measured from the TH images (green stars) overlaid on the waveguide dispersion that was measured by interferometric methods. The coloured arrows correspond to the four different wavelengths probed on Figs 5a,b and 6a , while the grey areas indicate the bandwidth associated with the 2.5 ps pulses. Full size image In the present demonstration, the key component—the waveguide-based time-to-space mapping element—is the PhC waveguide, which is ultra-compact (<100 μm long) and integrated on a chip. A fully integrated optical auto-correlator could be achieved by integrating a 3 dB splitter as well as the visible imaging system on-chip, thereby replacing the external lens/CCD camera. To accomplish this, our device could be integrated on top of a silicon-based linear detector array that would collect the THG signal directly in the near-field of the PhC waveguide, without lens assistance. Since the generated TH light is in the visible wavelength, it is therefore detectable with standard silicon detectors. The successful integration of near-infrared SWIFT spectrometers with a complicated set of sensitive single-photon detectors [38] points to the feasibility of this approach. This would yield a fully integrated device fabricated with solely CMOS technology, and without the need for any external instrumentation. The use of integrated detector arrays may also greatly improve the detection efficiency, allowing us to lower the required peak power level in the sub-watt regime, potentially down to the 10’s of milliwatt regime. A full analysis of the integrated detector sensitivity and resulting temporal resolution, however, lies outside the scope of this paper. Finally, it should be mentioned that, unlike SPIDER for example, the present device does not recover the phase information of the pulse. While in many cases the auto-correlation pulse shape is sufficient, the device performance could be further enhanced by exploiting on-chip pulse compression techniques [39] that provide a shorter reference pulse from the signal pulse itself to generate the spatial pulse intensity profile directly rather than the auto-correlation. While the performance of our device is not quite that of a commercial bulk-optics-based auto-correlator—our temporal resolution is slightly larger (~20 versus 5 fs for FR-103XL by Femtochrome) while our time window is slightly less (~20 versus 90 ps)—the compact nature and potential for full integration are major advantages that will enable many new applications. We also note that our performance can be improved by adopting different designs. For example, the 17 ps window can be extended up to 340 ps using a 2-mm-long integrated waveguide without degradation of the temporal resolution (see Methods). An apparent drawback of this device may be its bandwidth or wavelength range (15 nm versus an octave for a commercial instrument). However, the extreme compactness of the slow-light waveguide—more than two orders of magnitude shorter than a typical centimetre scale commercial auto-correlator—allows, in principle, the integration (with no moving parts) of parallel devices at staggered wavelengths to cover any wavelength range of interest. The C-band, for example, could be entirely covered by splitting the signal across only two–three spectrally detuned slow-light PhC waveguides, with the CCD camera monitoring the auto-correlation signals produced by the adjacent waveguides simultaneously. The operation wavelength of the flat-band slow-light window can be indeed finely adjusted during the lithography process [17] . Further, integrating a wavelength-demultiplexing device or dispersive element such as an AWG (readily available with silicon photonics technology) with an array of PhC waveguides on a chip would allow the application of this device to WDM signals of up to 50 or more channels. In summary, we have demonstrated a THG-based optical auto-correlator that employs an integrated and ultra-compact slow-light silicon PhC waveguide of less than 100 μm in length. Picosecond pulses near 1,550 nm are imaged directly along the PhC waveguide, providing reliable and potentially single-shot measurements of the pulse. We also demonstrate that this technique can be used as a simple and effective in situ diagnostic tool to study the propagation dynamics of near-infrared pulses into slow-light photonic crystal waveguides. This demonstration opens the door to realizing fully integrated devices capable of measuring ultra-fast near-infrared pulses on a silicon chip. Device structure and fabrication The device was fabricated from a SOITEC silicon-on-insulator wafer by electron-beam lithography (hybrid ZEISS GEMINI 1530/RAITH ELPHY) and reactive-ion etching using a CHF 3 /SF 6 gas mixture. The silica layer under the PhC slab was selectively under-etched using a HF solution to leave the PhC section in a suspended silicon membrane. The two dimensional PhC structure consists of a triangular lattice of air holes with lattice constant a =404 nm and hole radius 116 nm (0.287 a ) etched into a 220-nm-thick silicon suspended membrane. A W1 linear waveguide is created by omitting a single row of holes along the ΓK direction. The total PhC waveguide length is 96 μm, and the lattice period of the first and last 10 periods is stretched by around 10% (to ~444 nm) parallel to the waveguide axis so as to enhance the coupling to the slow-light mode. The dispersion of the PhC waveguide is engineered by laterally shifting the first rows of holes adjacent to the waveguide centre in the direction perpendicular to the waveguide axis. For the dispersion-engineered waveguide used in this experiment, the rows closest to the centre are shifted 50 nm away from the axis of the waveguide and the mode effective area A eff is around 0.5 μm 2 . The PhC waveguide is connected on both sides to 200-μm-long access nanowires (220 nm × 700 nm cross-section) terminated by inverse tapers, and embedded into large mode area ( A eff ~8 μm 2 ) SU8 polymer waveguides to improve the coupling to the chip via butt-coupled lensed fibres. The total fibre-to-fibre transmission is about −9.5 dB in the present experiment. The absolute group velocity dispersion β 2 for the engineered fundamental PhC waveguide mode ranges between 3 × 10 −21 s 2 m −1 , in the flat-band slow-light window, up to 5 × 10 −20 s 2 m −1 in the dispersive band between 1,545 and 1,550 nm. This provides an associated dispersion length for 2.5 ps pulses between 125 μm and 2 mm. This is longer than the entire PhC waveguide length, so we expect the effect of dispersion on all our measurements to be negligible. In the flat-band slow-light window with reduced dispersion, this value of β 2 enables, in principle, the measurement of pulses as short as 550 fs without distortion along the waveguide. Such short pulses could be readily mapped along the length of our device since they would have a spatial extension within the waveguide of ~5.5 μm, which is ~14 times larger than the spatial resolution of our imaging set-up (see below). Optical testing As shown in Fig. 1 , the experimental set-up consists of splitting optical pulses (2.5 ps pulses at 10 MHz repetition rate, λ =1,550 nm, ~10 W peak power) from a tunable mode-locked fibre laser and launching the resulting counter-propagating replicas onto the chip. The two arms of the set-up include polarization controllers, attenuators and circulators to select the TE polarization and balance the optical power, measured onto power meters (through 1% couplers), arising from either side. We noticed that the TH pattern was not very sensitive in finding the perfect power balance though. One arm contains a motorized tunable delay line (with a maximum delay of 250 ps) to match the optical path lengths on both sides. Note that all of these components could be avoided with the use of an integrated 3 dB splitter. The average power launched on each side of the chip for the auto-correlation measurement presented in Fig. 3 (at 1,548 nm, n g ~23) is about 200 μW, corresponding to around ~3.2 W coupled peak power for −4 dB estimated insertion loss. When tuning the signal wavelength as in Figs 5 , 6 to explore the impact of the group velocity while maintaining a THG-based auto-correlation trace with a relatively high signal-to-noise ratio, the input power was slightly varied from 2 to 3.5 W coupled peak power. This was done to compensate for (1) the decrease of the THG efficiency at lower group indices [22] , (2) the slight increase in the propagation loss with the group index and (3) the decrease in the collection efficiency of the cross-THG signal for increasing wavevectors (that is, larger wavelengths). A 0.65 NA Mitutoyo objective is used to collect the TH signal emitted from the top of the PhC waveguide and imaged onto a high-resolution silicon CCD visible camera. A beam splitter complements the free-space optic collection system to simultaneously image the waveguide in the Fourier plane on another visible CCD camera. The details on the Fourier-space measurements are further explained in Monat et al . [32] For the figures displaying the profile of the TH intensity, the TH signal is averaged over 17 pixels in the lateral direction centred on the waveguide axis. Time-to-space mapping and device resolution Our auto-correlator device effectively provides a time ( T )-to-space ( Z coordinate along the waveguide axis) mapping of the pulse temporal characteristics through the following relation: T = Z × c / n g when accounting for the group velocity c / n g of the pulse into the PhC waveguide. In addition, the cross-THG intensity image provides a temporal profile that is compressed by a factor √3 with respect to the pulse intensity profile, as estimated from numerical simulations of the THG produced by the sum of the left and right electric field and integrated over the pulse duration. With our observation system (lens and CCD camera), the distance between the conjugate points of the PhC waveguide imaged by adjacent pixels is ~0.14 μm. However, for our off-chip imaging system, the actual spatial resolution is given by the diffraction limit, that is, ~ λ /(2 × NA), resulting in ~400 nm for the TH signal detected at 520 nm and the objective (NA=0.65) used here. Note that this roughly corresponds to the period of the PhC, which eventually limits the attainable resolution due to the Bloch mode nature of the underlying PhC waveguide mode that produces THG. This translates into ~53 fs (69 fs) temporal resolution for the pulse duration when considering a group velocity of c /23 ( c /30), as used in this particular device. Note that the temporal resolution and maximum pulse duration that can be measured with our device, respectively, decrease and increase with the group index of the waveguide, as illustrated in Table 1 . The longest pulse duration or time window mapped into space to be measured with the device can be readily extended by increasing the PhC waveguide length to the extent of dispersion remaining negligible, that is, up to 340 ps for a 2-mm-long PhC waveguide (in the c /30 flat-band slow-light window). The shortest pulse duration available to measurement is primarily governed by the dispersion length of the PhC waveguide, that is, here 550 fs, rather than the time resolution provided by our device. For the equivalent of ‘time-of-flight measurements’ in Fig. 6 , the tunable delay line is scanned across ~10 ps, so as to change the crossing point location within the waveguide, where the right and left pulses do meet. Tracking the TH profile centre location versus the delay gives a linear curve. The slope is equal to half of the group velocity, since the crossing point moves twice as slow as the pulses. This allows us to extract the average group velocity at which the pulse propagates without any assumption or fit parameter, and with a resolution limited by diffraction. How to cite this article: Monat, C. et al . Integrated optical auto-correlator based on third-harmonic generation in a silicon photonic crystal waveguide. Nat. Commun. 5:3246 doi: 10.1038/ncomms4246 (2014).